The acetyltransferase HAT1 moderates the NF-κB response by regulating the transcription factor PLZF To date, the activities of protein kinases have formed the core of our understanding of cell signal transduction. Comprehension of the extent of protein acetylation has raised expectations that this alternate post-transcriptional modification will be shown to rival phosphorylation in its importance in mediating cellular responses. However, limited instances have been identified. Here we show that signalling from Toll-like or TNF-α receptors triggers the calcium/calmodulin-dependent protein kinase (CaMK2) to activate histone acetyltransferase-1 (HAT1), which then acetylates the transcriptional regulator PLZF. Acetylation of PLZF promotes the assembly of a repressor complex incorporating HDAC3 and the NF-κB p50 subunit that limits the NF-κB response. Accordingly, diminishing the activity of CaMK2, the expression levels of PLZF or HAT1, or mutating key residues that are covalently modified in PLZF and HAT1, curtails control of the production of inflammatory cytokines. These results identify a central role for acetylation in controlling the inflammatory NF-κB transcriptional programme. Post-translational modifications of amino acids are critical to regulate enzyme activity. Of the numerous covalent modifications, the consequence of protein phosphorylation has been most prominent and it forms the core of our understanding of how cell signal transduction mediates biological responsiveness. Recent proteomic analysis has shown that the extent of acetylation approaches that observed for phosphorylation [1] , suggesting that this covalent modification is also highly influential in regulating cellular processes. However, there are limited expositions of the consequences of acetylation of non-histone substrates. Here, by probing innate immune cell signalling pathways triggered by Toll-like (TLR) and tumour necrosis factor receptors (TNFR), we show that the ensuing nuclear factor kappa-light-chain-enhancer of activated B cells (NF-κB)-dependent inflammatory response depends upon acetylation by the type-B histone acetylase-1 (HAT1). Inflammatory responses are critical to survival and must be tightly regulated to ensure appropriate immune protection without damage to the host. The inducible NF-κB response instigates the primary transcriptional response to a broad range of infectious stimuli. Unremitting NF-κB activity in many pathological conditions has marked it as a major therapeutic target. However, general inhibitors of the NF-κB pathway have had confounding and even detrimental effects. Promisingly, analysis of transcripts induced during the innate immune response demonstrates distinct regulation of functional gene subsets [2] . This specificity is afforded via distinct transcription complexes that alternately promote or repress select genes. Identifying the specific components of functionally distinct transcriptional complexes is essential to inform a rational therapeutic strategy against damaging innate immune responses. Towards this, we identify the transcriptional regulator promyelocytic leukaemia zinc finger protein (PLZF) as a critical co-factor of the NF-κB transcriptional complex that limits damaging inflammation. PLZF belongs to the Broad-complex, Tramtrack and Bric-a-brac (BTB)/poxvirus and zinc finger family of transcription factors that regulate a variety of biological processes, including development, differentiation, tumourigenesis and, as is emerging, the immune response [3] . PLZF functions as a transcriptional regulator by binding to a specific motif in gene promoters, via its C-terminal Krueppel-type zinc-finger domains, and recruits transcription co-factors, via its N-terminal BTB domain. The protein functions as either a transcriptional repressor or inducer, depending on different covalent modifications [4] . We identify that, following TLR and TNFR signalling, PLZF forms a novel repressor complex consisting of histone deacetylase 3 (HDAC3) and the NF-κB p50 subunit, thereby suppressing the production of NF-κB-induced inflammatory cytokines. Importantly, we identify that the formation of this critical repressor complex is brought about by acetylation of PLZF by HAT1. HAT1 was the very first histone acetyltransferase to be identified. The enzyme was previously established to acetylate newly synthesized cytoplasmic histones (specifically H3 and H4). As such, HAT1 is important in replication-dependent chromatin assembly. The enzyme has also been shown to participate in DNA repair and telomeric gene silencing. Here we identify that HAT1 is activated during innate immune signalling through the activity of the calcium/calmodulin-dependent protein kinase (CaMK2), to acetylate PLZF. This covalent modification is required for assembly of the PLZF, HDAC3 and NF-κB p50 repressor complex. Accordingly, HAT1 activity is required for correct regulation of the NF-κB transcriptional programme. This unconventional role for HAT1 identifies a novel role for acetyltransferases in cell signalling that is critical for the innate immune response. PLZF limits endotoxic shock Previously, we identified the transcription factor PLZF as a positive regulator of interferon (IFN)-regulated gene expression induced during the antiviral response [5] . To determine the physiological consequences of PLZF function in the immediate innate immune response, we compared the survival of wild-type (WT) and PLZF-deficient ( Zbtb16 −/− ) mice injected with the TLR4 ligand lipopolysaccharide (LPS). The results ( Fig. 1a ) showed that PLZF-deficient mice were more susceptible to endotoxic shock, suffering a significantly higher mortality than WT mice. Analysis of circulating inflammatory cytokine levels at early times after LPS injection showed that levels of tumour necrosis factor α (TNF-α), interleukin (IL)-6 and IL-12 were significantly elevated in the PLZF-deficient mice ( Fig. 1b ). Consistent with this, the levels of the Il-6 , Il-12 and Tnf-α transcripts were more induced in bone marrow-derived macrophages (BMMs) from Zbtb16 −/− compared to WT mice treated with LPS ( Fig. 1c ). These data show that PLZF represses the inflammatory response. 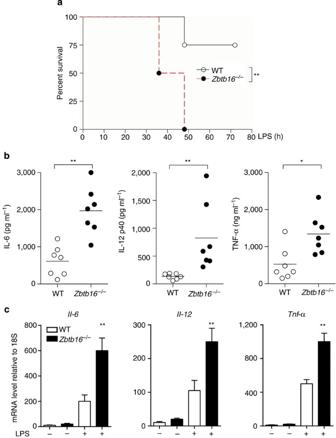Figure 1: PLZF limits endotoxic shock. (a) Comparison of the relative survival of WT andZbtb16−/−mice injected with LPS (20 mg kg−1; Wilcoxon test, **P<0.01,n=7 per group). (b) The levels of IL-6, IL-12 and TNF-α in serum taken from endotoxin-challenged WT andZbtb16−/−mice after 2 h. Data are representative of repeated independent experiments and show the means±s.d. of three replicates. *P<0.05, **P<0.01, by Student’st-test. (c) The levels of theIl-6,Il-12andTnf-αmRNAs that were induced in BMM taken from WT andZbtb16−/−mice after stimulus with LPS (100 ng ml−1) for 30 min. Figure 1: PLZF limits endotoxic shock. ( a ) Comparison of the relative survival of WT and Zbtb16 −/− mice injected with LPS (20 mg kg −1 ; Wilcoxon test, ** P <0.01, n =7 per group). ( b ) The levels of IL-6, IL-12 and TNF-α in serum taken from endotoxin-challenged WT and Zbtb16 −/− mice after 2 h. Data are representative of repeated independent experiments and show the means±s.d. of three replicates. * P <0.05, ** P <0.01, by Student’s t -test. ( c ) The levels of the Il-6 , Il-12 and Tnf-α mRNAs that were induced in BMM taken from WT and Zbtb16 −/− mice after stimulus with LPS (100 ng ml −1 ) for 30 min. Full size image PLZF suppresses NF-κB transactivation We probed the TLR signalling pathway in order to identify the point at which PLZF functions. The data showed that the hyper-responsiveness of Zbtb16 −/− cells was not due to increased receptor-proximal signalling, as the activation kinetics of the signalling molecules, pERK, p38 MAPK, JNK and NF-κB, were equivalent between the WT and Zbtb16 −/− BMMs ( Fig. 2a ). Despite this, an electrophoretic mobility shift assay (EMSA) detected enhanced DNA binding by the NF-κB complex in Zbtb16 −/− BMMs ( Fig. 2b ). Quantification of the NF-κB subunits, by ELISA, demonstrated that this was due to increased p65 binding in lysates of Zbtb16 −/− compared with WT BMMs stimulated with LPS ( Fig. 2c ). 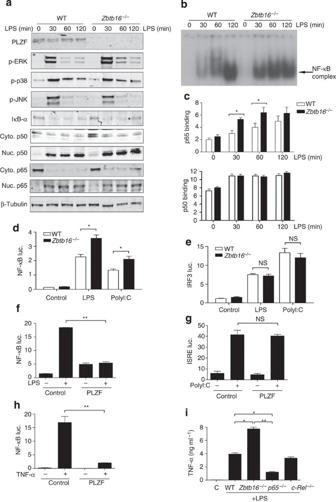Figure 2: PLZF suppresses NF-κB transactivation. (a) Immunoblots detecting the activation kinetics of the indicated signalling molecules in lysates from the whole cell, cytosol (Cyto.) or nucleus (Nuc.) from WT orZbtb16−/−BMMs treated with LPS (100 ng ml−1). (b) Enhanced binding of a32P-labelled oligonucleotide containing an NF-κB recognition element in nuclear extracts fromZbtb16−/−compared with WT BMMs treated with LPS (100 ng ml−1) for the indicated times. (c) The relative binding of the NF-κB p50 and p65 subunits to the oligonucleotide containing an NF-κB recognition element in nuclear extracts fromZbtb16−/−compared with WT BMMs treated as inb. (d,e) Increased NF-κB activity inZbtb16−/−compared with WT BMMs detected by the activity of NF-κB- or, as a control, IRF3-responsive firefly luciferase (luc.) reporter plasmids after treatment for 4 h with LPS (100 ng ml−1) or polyI:C (10 μg ml−1). (f,g) Luciferase activity in TLR4- or TLR3-HEK293T cells transfected with NF-κB- or, as a control, interferon-stimulated response element-responsive firefly luciferase reporter and empty or PLZF-expressing plasmids after stimulation with LPS (10 ng ml−1) or polyI:C (25 μg ml−1). (h) Luciferase activity in HEK293T cells transfected with NF-κB-responsive reporters and empty or PLZF-expressing plasmids, then stimulated with TNF-α (10 ng ml−1). (i) The levels of TNF-α measured by ELISA in supernatants from BMMs of WT,RelA−/−(p65−/−),c-Rel−/−andZbtb16−/−mice stimulated with LPS (100 ng ml−1) for 6 h. See alsoSupplementary Fig. 1a–c. All experimentsn⩾3, bars represent mean±s.d. *P<0.05, **P<0.01 and not significant (NS) by Student’st-test. Figure 2: PLZF suppresses NF-κB transactivation. ( a ) Immunoblots detecting the activation kinetics of the indicated signalling molecules in lysates from the whole cell, cytosol (Cyto.) or nucleus (Nuc.) from WT or Zbtb16 −/− BMMs treated with LPS (100 ng ml −1 ). ( b ) Enhanced binding of a 32 P-labelled oligonucleotide containing an NF-κB recognition element in nuclear extracts from Zbtb16 −/− compared with WT BMMs treated with LPS (100 ng ml −1 ) for the indicated times. ( c ) The relative binding of the NF-κB p50 and p65 subunits to the oligonucleotide containing an NF-κB recognition element in nuclear extracts from Zbtb16 −/− compared with WT BMMs treated as in b . ( d , e ) Increased NF-κB activity in Zbtb16 −/− compared with WT BMMs detected by the activity of NF-κB- or, as a control, IRF3-responsive firefly luciferase (luc.) reporter plasmids after treatment for 4 h with LPS (100 ng ml −1 ) or polyI:C (10 μg ml −1 ). ( f , g ) Luciferase activity in TLR4- or TLR3-HEK293T cells transfected with NF-κB- or, as a control, interferon-stimulated response element-responsive firefly luciferase reporter and empty or PLZF-expressing plasmids after stimulation with LPS (10 ng ml −1 ) or polyI:C (25 μg ml −1 ). ( h ) Luciferase activity in HEK293T cells transfected with NF-κB-responsive reporters and empty or PLZF-expressing plasmids, then stimulated with TNF-α (10 ng ml −1 ). ( i ) The levels of TNF-α measured by ELISA in supernatants from BMMs of WT, RelA −/− ( p65 −/− ), c-Rel −/− and Zbtb16 −/− mice stimulated with LPS (100 ng ml −1 ) for 6 h. See also Supplementary Fig. 1a–c . All experiments n ⩾ 3, bars represent mean±s.d. * P <0.05, ** P <0.01 and not significant (NS) by Student’s t -test. Full size image The effect of PLZF on NF-κB activity was further measured using NF-κB-responsive luciferase reporters. PLZF was demonstrated to repress an NF-κB-, and not an IFN regulatory factor 3 (IRF3)-, regulated luciferase reporter in WT and Zbtb16 −/− BMMs stimulated with LPS or polyinosinic-polycytidylic acid (polyI:C; Fig. 2d,e ). Similarly, PLZF repressed an NF-κB-, and not an IFN-stimulated response element-, regulated reporter in HEK293T cells expressing either TLR4, MD2 and CD14, or TLR3 (TLR3/4-HEK293T [6] ) stimulated with LPS or polyI:C ( Fig. 2f,g ). This effect was not restricted to TLR signalling, as demonstrated by PLZF-dependent repression of NF-κB activity after TNF-α stimulation ( Fig. 2h ). Consistent with these data, the induction of TNF-α and IL-6 was attenuated in NF-κB p65 (RelA) ablated, but remained largely unaltered in c-Rel ablated, macrophages ( Fig. 2i and Supplementary Fig. 1a ). Similarly, the enhanced induction of TNF-α in Zbtb16 −/− and WT BMMs was attenuated with an NF-κB inhibitor (BAY11-7085; Supplementary Fig. 1b ). There was also an enhanced association of PLZF with an Il-6 promoter reporter upon treatment with LPS ( Supplementary Fig. 1c ). These data demonstrate that PLZF represses NF-κB transactivation. Formation of the repressor complex is regulated by acetylation of PLZF As the repressor function of PLZF is reportedly regulated by acetylation, albeit that the residues previously identified are peripheral to the activity identified here [7] , we probed the acetylation status of FLAG-PLZF overexpressed in TLR4-HEK293T cells treated with LPS by immunoprecipitation (IP) and western blot. The data showed that PLZF was acetylated upon treatment with LPS ( Fig. 3a ). The TLR-stimulus-dependent acetylation of endogenously expressed PLZF was confirmed in WT and Zbtb16 −/− BMM ( Fig. 3b ). Computational analysis (using the ASEB and PHOSIDA web servers) identified two putative acetylation sites, at the lysine residue numbers 271 and 277, within the repressor domain (RD) of PLZF ( Supplementary Table 1 ). Substituting glutamine, arginine or similarly alanine, by point mutagenesis (to mimic the respective acetylated or non-acetylated states) tested the significance of these lysine residues. These data revealed that the K277 residue was acetylated ( Fig. 3c,d and Supplementary Fig. 2a ). In addition, the K277 residue was demonstrated to be required for repression of NF-κB activity in LPS- and TNF-α-stimulated TLR4-HEK293T cells ( Fig. 3e and Supplementary Fig. 2b–e ). Moreover, we demonstrated that the normal control of cytokine production could be restored in Zbtb16 −/− BMM by transformation with retrovirus that expressed WT but not mutant PLZF (K271R+K277R; Fig. 3f and Supplementary Fig. 2f ). These data identified that the PLZF-dependent repression of NF-κB activity requires acetylation of the K277 residue. 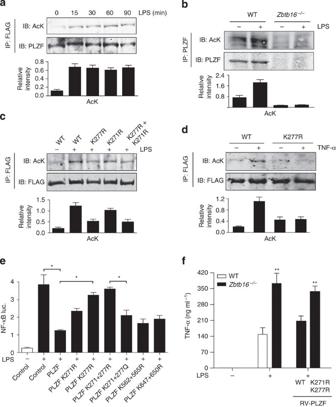Figure 3: Acetylation of PLZF regulates NF-κB activity. (a) Detection of PLZF acetylation in TLR4-HEK293 cells transiently transfected with FLAG-PLZF and treated with LPS (100 ng ml−1) for the indicated times. Whole-cell lysates were IP with anti-FLAG and proteins detected by immunoblot (IB) with anti-acetylated-lysine (AcK) and -PLZF antibodies. (b) Detection of the acetylation of endogenous PLZF in WT andZbtb16−/−BMM treated with LPS (10 ng ml−1) for 30 min, then whole-cell lysates were IP with anti-PLZF and enriched proteins probed by IB with anti-AcK antibodies. (c,d) Identification of acetylated lysine residues on PLZF from HEK293T or TLR4-HEK293T cells transiently transfected with FLAG-tagged WT or the indicated mutant PLZF expression plasmids, followed by treatment for 30 min with LPS (100 ng ml−1) or TNF-α (10 ng ml−1). The proteins were enriched from whole-cell lysates by IP then detected by IB with the indicated antibodies. See alsoSupplementary Fig 2a. The extent of PLZF acetylation is quantified in the graphs below (a–d). (e) Evaluation of the dependence of specific lysines on PLZF to luciferase activity in TLR4-HEK293T cells co-transfected with NF-κB-responsive firefly and empty vector (Control) or PLZF constructs as labelled after treatment for 5 h with LPS (100 ng ml−1). See alsoSupplementary Fig. 2b–e. (f) TNF-α production measured by ELISA by WT andZbtb16−/−BMM transformed with retrovirus (RV-PLZF) expressing WT of mutant (K271R+K277R) PLZF then treated with LPS for 30 min. See alsoSupplementary Fig. 2f. All experimentsn⩾3, bars represent mean±s.d. *P<0.05, **P<0.01 by Student’st-test. Figure 3: Acetylation of PLZF regulates NF-κB activity. ( a ) Detection of PLZF acetylation in TLR4-HEK293 cells transiently transfected with FLAG-PLZF and treated with LPS (100 ng ml −1 ) for the indicated times. Whole-cell lysates were IP with anti-FLAG and proteins detected by immunoblot (IB) with anti-acetylated-lysine (AcK) and -PLZF antibodies. ( b ) Detection of the acetylation of endogenous PLZF in WT and Zbtb16 −/− BMM treated with LPS (10 ng ml −1 ) for 30 min, then whole-cell lysates were IP with anti-PLZF and enriched proteins probed by IB with anti-AcK antibodies. ( c , d ) Identification of acetylated lysine residues on PLZF from HEK293T or TLR4-HEK293T cells transiently transfected with FLAG-tagged WT or the indicated mutant PLZF expression plasmids, followed by treatment for 30 min with LPS (100 ng ml −1 ) or TNF-α (10 ng ml −1 ). The proteins were enriched from whole-cell lysates by IP then detected by IB with the indicated antibodies. See also Supplementary Fig 2a . The extent of PLZF acetylation is quantified in the graphs below ( a – d ). ( e ) Evaluation of the dependence of specific lysines on PLZF to luciferase activity in TLR4-HEK293T cells co-transfected with NF-κB-responsive firefly and empty vector (Control) or PLZF constructs as labelled after treatment for 5 h with LPS (100 ng ml −1 ). See also Supplementary Fig. 2b–e . ( f ) TNF-α production measured by ELISA by WT and Zbtb16 −/− BMM transformed with retrovirus (RV-PLZF) expressing WT of mutant (K271R+K277R) PLZF then treated with LPS for 30 min. See also Supplementary Fig. 2f . All experiments n ⩾ 3, bars represent mean±s.d. * P <0.05, ** P <0.01 by Student’s t -test. Full size image The acetyltransferase HAT1 controls PLZF activity Next we tried to identify the acetyltransferase that modifies PLZF. Although CBP/p300 had previously been demonstrated to acetylate the C-terminus of PLZF [7] , it did not affect PLZF-dependent regulation of an NF-κB reporter plasmid ( Supplementary Fig. 3a ). As PLZF had previously been identified to interact with the type B histone acetyltransferase HAT1 (ref. 8 ), and because the residues surrounding K277 of PLZF accords with a HAT1 substrate-specific motif (GxGKxG [9] ; Supplementary Table 1 ), we tested a role for HAT1 in PLZF-dependent inhibition of NF-κB transactivation. To begin with, we confirmed the proteins associated by co-immunoprecipitation (co-IP) of HAT1 and PLZF overexpressed in HEK293T cells ( Fig. 4a ). An association between the endogenous proteins was confirmed in WT and Zbtb16 −/− BMM ( Fig. 4b ). Next, we showed that reduced expression of HAT1 in HEK293T cells expressing a short hairpin (sh) RNA ablated TNF-α-induced acetylation of PLZF ( Fig. 4c ). Furthermore, knocking down HAT1 expression ablated PLZF-dependent repression of an NF-κB reporter in HEK293T cells stimulated with TNF-α ( Fig. 4d ). Strikingly, knocking down HAT1 or PLZF expression in the human monocytic cell line, THP1, led to equivalent, excess production of TNF-α in response to the TLR7 ligand imiquimod ( Fig. 4e and Supplementary Fig. 3b,c ). 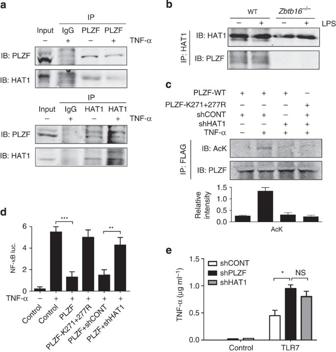Figure 4: The acetyltransferase HAT1 controls PLZF activity. (a) Detection of an interaction between HAT1 and PLZF expressed in HEK293T cells treated for 30 min with TNF-α by IP from whole-cell lysates followed by immunoblot (IB) with the indicated antibodies. IgG is used as a control for the specificity of the IP. (b) Detection of an interaction between endogenous HAT1 and PLZF in WT, and as a controlZbtb16−/−BMM by IP then IB with the indicated antibodies. (c) Detection of HAT1-dependent acetylation of PLZF from HEK293T cells co-transfected with control (shCONT) or HAT1 (shHAT1) targeting shRNAs and WT or mutant (K271/277R) PLZF-expressing plasmids, followed by treatment for 30 min with TNF-α (10 ng ml−1). Whole-cell lysates were IP and IB with the indicated antibodies. The extent of PLZF acetylation is quantified in the graph below. (d) Detection of HAT1-dependent regulation of NF-κB activity by luciferase assay in HEK293T cells co-transfected with NF-κB-responsive firefly and control or HAT1 targeting shRNAs and WT or mutant (K271/277R) PLZF constructs, after stimulation with TNF-α (10 ng ml−1) for 5 h. (e) The levels of TNF-α production by THP1 cells expressing control (shCONT), PLZF (shPLZF) or HAT1 (shHAT1) targeting shRNA treated with the TLR7 ligand imiquimod (10 μg ml−1) for 5 h. Also seeSupplementary Fig. 3b and c. All experimentsn⩾3, bars represent mean±s.d. *P<0.05, **P<0.01, ***P<0.001 and not significant (NS) by Student’st-test. Figure 4: The acetyltransferase HAT1 controls PLZF activity. ( a ) Detection of an interaction between HAT1 and PLZF expressed in HEK293T cells treated for 30 min with TNF-α by IP from whole-cell lysates followed by immunoblot (IB) with the indicated antibodies. IgG is used as a control for the specificity of the IP. ( b ) Detection of an interaction between endogenous HAT1 and PLZF in WT, and as a control Zbtb16 −/− BMM by IP then IB with the indicated antibodies. ( c ) Detection of HAT1-dependent acetylation of PLZF from HEK293T cells co-transfected with control (shCONT) or HAT1 (shHAT1) targeting shRNAs and WT or mutant (K271/277R) PLZF-expressing plasmids, followed by treatment for 30 min with TNF-α (10 ng ml −1 ). Whole-cell lysates were IP and IB with the indicated antibodies. The extent of PLZF acetylation is quantified in the graph below. ( d ) Detection of HAT1-dependent regulation of NF-κB activity by luciferase assay in HEK293T cells co-transfected with NF-κB-responsive firefly and control or HAT1 targeting shRNAs and WT or mutant (K271/277R) PLZF constructs, after stimulation with TNF-α (10 ng ml −1 ) for 5 h. ( e ) The levels of TNF-α production by THP1 cells expressing control (shCONT), PLZF (shPLZF) or HAT1 (shHAT1) targeting shRNA treated with the TLR7 ligand imiquimod (10 μg ml −1 ) for 5 h. Also see Supplementary Fig. 3b and c . All experiments n ⩾ 3, bars represent mean±s.d. * P <0.05, ** P <0.01, *** P <0.001 and not significant (NS) by Student’s t -test. Full size image The kinase CaMK2 activates HAT1 We sought to identify how HAT1 was activated during the innate immune response. As a proteomic screen had previously identified that HAT1 was phosphorylated at the serine residue number 361 within a putative CaMK2 substrate motif [10] , and because CaMK2 controls NF-κB activity during the innate immune reaction [11] , [12] , we tested if CaMK2 affected HAT1 activation in HEK293 cells expressing WT and mutant protein constructs. This experiment demonstrated that HAT1 was acetylated by treatment with TNF-α, confirming activation of the acetyltransferase during innate immune cell signalling ( Fig. 5a ). A role for the HAT1 phosphor-S361 residue in innate immune signalling was supported by the demonstration that a mutant HAT1 (S361A) remained unacetylated in this experiment. Significantly, inhibiting CaMK2 activity with a methoxybenzenesulfonamide inhibitor (KN-93) reduced HAT1 acetylation in this experiment ( Fig. 5a and Supplementary Fig. 4a ). This activity was confirmed for the endogenous proteins by measuring HAT1 acetylation in THP-1 cells with CaMK2 expression repressed by RNA interference ( Fig. 5b and Supplementary Fig. 4b,c ). We tested if the association between endogenous PLZF and HAT1 required CaMK2 activity in THP-1 cells expressing control or CaMK2-targeting shRNAs by in situ proximity ligation assay (PLA). Resting control cells (shCONT) showed a marked increase in foci, corresponding to complexes of PLZF and HAT1, which was ablated in cells with reduced CaMK2 expression (shCaMK2) upon TNF-α stimulation ( Fig. 5c ). This experiment identified an enhanced association between PLZF and HAT1 after stimulus that was not apparent by co-IP. This pathway was further tested by measuring the expression of an NF-κB-dependent reporter in HEK293T cells treated with TNF-α and expressing WT or lysine mutant PLZF, and with HAT1 expression either reduced by RNA interference or elevated by expression of the WT or the phosphor-residue mutant (S361A) HAT1. 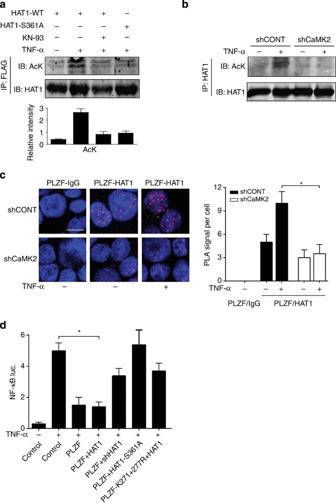Figure 5: HAT1 activity is regulated by CaMK2. (a) Detection of CaMK2-dependent activation of HAT1 by measuring HAT1 acetylation in HEK293T cells transfected with WT or mutant (S361A) FLAG-HAT1 expression plasmids, treated for 30 min with TNF-α (10 ng ml−1) and a CaMK2 inhibitor (KN-93). Whole-cell lysates were IP and immunoblotted (IB) with the indicated antibodies. The extent of HAT1 acetylation is quantified in the graph below the IB. Also seeSupplementary Fig. 4a. (b) Detection of CaMK2-dependent activation of endogenous HAT1 by measuring HAT1 acetylation in THP-1 cells expressing control (shCONT) or CaMK2-targeting (shCaMK2) shRNAs and treated with TNF-α for 30 min. Whole-cell lysates were IP and IB with the indicated antibodies. Also seeSupplementary Fig. 4b and c. (c) Micrographs showing the interaction between endogenous PLZF and HAT1 as red foci in control (shCONT) or CaMK2-knockdown (shCaMK2) THP-1 cells treated with TNF-α (10 ng ml−1) for 30 min. IgG are used as controls. The graph to the right of the micrographs shows a quantification of the protein interactions detected by PLA from 200 cells (using OLINK). Cell nuclei are stained blue by Hoechst dye (scale bar, 10 μm). (d) Evaluation of the requirement of HAT1 itself and the serine residue number 361 of HAT1 for the PLZF-dependent repression by measuring luciferase activity in HEK293T cells transfected with an NF-κB-responsive reporter and empty vector (Control), PLZF and either WT or mutant (S361A) HAT1, or an shRNA targeting HAT1 and treated with TNF-α (10 ng ml−1) for 5 h. All experimentsn⩾3, bars represent mean±s.d. *P<0.05 by Student’st-test. Figure 5d demonstrates that PLZF-dependent control of NF-κB activity requires the WT HAT1 protein. Figure 5: HAT1 activity is regulated by CaMK2. ( a ) Detection of CaMK2-dependent activation of HAT1 by measuring HAT1 acetylation in HEK293T cells transfected with WT or mutant (S361A) FLAG-HAT1 expression plasmids, treated for 30 min with TNF-α (10 ng ml −1 ) and a CaMK2 inhibitor (KN-93). Whole-cell lysates were IP and immunoblotted (IB) with the indicated antibodies. The extent of HAT1 acetylation is quantified in the graph below the IB. Also see Supplementary Fig. 4a . ( b ) Detection of CaMK2-dependent activation of endogenous HAT1 by measuring HAT1 acetylation in THP-1 cells expressing control (shCONT) or CaMK2-targeting (shCaMK2) shRNAs and treated with TNF-α for 30 min. Whole-cell lysates were IP and IB with the indicated antibodies. Also see Supplementary Fig. 4b and c . ( c ) Micrographs showing the interaction between endogenous PLZF and HAT1 as red foci in control (shCONT) or CaMK2-knockdown (shCaMK2) THP-1 cells treated with TNF-α (10 ng ml −1 ) for 30 min. IgG are used as controls. The graph to the right of the micrographs shows a quantification of the protein interactions detected by PLA from 200 cells (using OLINK). Cell nuclei are stained blue by Hoechst dye (scale bar, 10 μm). ( d ) Evaluation of the requirement of HAT1 itself and the serine residue number 361 of HAT1 for the PLZF-dependent repression by measuring luciferase activity in HEK293T cells transfected with an NF-κB-responsive reporter and empty vector (Control), PLZF and either WT or mutant (S361A) HAT1, or an shRNA targeting HAT1 and treated with TNF-α (10 ng ml −1 ) for 5 h. All experiments n ⩾ 3, bars represent mean±s.d. * P <0.05 by Student’s t -test. Full size image These data demonstrate that activation of HAT1 and this protein’s association with PLZF, and the ensuing repression of NF-κB activity depended on the S361 phosphor-residue of HAT1 and required CaMK2 activity. PLZF recruits HDAC3 and NF-κB p50 to repress NF-κB activity We next sought to define the mechanism by which PLZF controls the levels of inflammatory cytokines. To do this, we mapped the regions of PLZF that repressed NF-κB transcriptional activity using a series of truncated PLZF mutants ( Supplementary Fig. 5 ) expressed in the TLR4-HEK293T cells. The data indicated that the central repressor (RD) and bric-a-brac, tramtrack and broad complex (BTB) domains of PLZF were sufficient to mediate repression ( Fig. 6a ). Since the DNA-binding function of PLZF is dispensable for repression, this ruled out direct tethering to promoters and suggests that PLZF negatively regulates NF-κB-mediated transactivation entirely by recruiting transcription co-factors. In light of this and because PLZF had been reported to interact with HDACs that form a transcriptional repressor complex with NF-κB p50 (refs 13 , 14 , 15 , 16 ), we tested if PLZF repressed NF-κB transcription activity through an association with NF-κB p50 and/or HDACs. Overexpression of NF-κB p50 or HDAC3, and to a lesser extent HDAC1, repressed LPS-stimulated NF-κB activity in TLR4-HEK293T cells ( Fig. 6b ). The inhibitory effect of HDAC3 required its deacetylase activity, as a catalytically inactive HDAC3 mutant (Y298H) was unable to inhibit NF-κB activity ( Fig. 6c ) [17] . Moreover, combined overexpression of PLZF, NF-κB p50 and HDAC3 shows that these factors function co-ordinately to repress NF-κB activity ( Fig. 6d ). 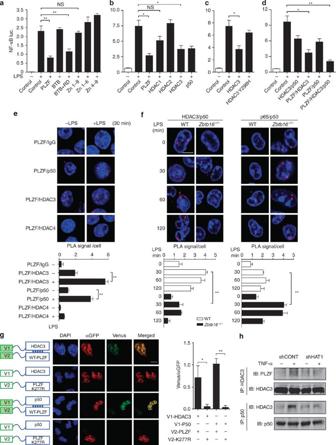Figure 6: The BTB and repressor domains of PLZF recruit HDAC3 and NF-κB p50 to repress NF-κB activity. (a–d) Luciferase activity in TLR4-HEK293T cells stimulated for 5 h with LPS (10 ng ml−1), 24 h after co-transfection with NF-κB-responsive reporters and: (a) empty (Control) or the indicated truncated PLZF constructs. See alsoSupplementary Fig. 5; (b) PLZF, HDAC1, HDAC2, HDAC3 or NF-κB p50 expression constructs; (c) WT or catalytically inactive HDAC3 (Y298H); and (d) HDAC3 with NF-κB p50, or PLZF, and all three protein expression constructs combined. (e,f) Micrographs showing the interaction between endogenous PLZF and HDAC3 or NF-κB p50 and HDAC3 with p50 or p65 detected as red foci in (e) RAW264.7 cells, or (f) WT andZbtb16−/−BMMs stimulated with LPS (100 ng ml−1). Graphs below show a quantitation of the protein interactions detected by PLA from 200 cells (using OLINK). HDAC4 and the IgG are used as controls. Cell nuclei are stained blue by Hoechst dye (scale bar, 10 μm). (g) Detection of the dependence of the K277 residue of PLZF for protein association by BiFl using HEK293T cells transfected with WT or mutant (K277R) PLZF tagged with the V2 split Venus fluorophore and either NF-κB p50 or HDAC3 fused with the alternate V1 half of Venus (scale bar, 10 μm). Expression of PLZF is confirmed with an antibody (αGFP) to V2 and used to normalize the level of Venus fluorescence to protein expression in the graph to the right of the micrographs. The complexes being detected are depicted in the schematic shown on the left of the micrographs. (h) Demonstration of the dependence of HAT1 expression for the formation of the co-repressor protein complex, by detecting the association between HDAC3 and PLZF, or NF-κB p50 through IP and immunoblot (IB) with the indicated antibodies in THP-1 cells expressing a control (shCONT) orHAT1-targeting (shHAT1) shRNAs treated with TNF-α (10 ng ml−1) for 30 min. All experimentsn⩾3, bars represent mean±s.d. *P<0.05, **P<0.01, and not significant (NS) by Student’st-test. Figure 6: The BTB and repressor domains of PLZF recruit HDAC3 and NF-κB p50 to repress NF-κB activity. ( a – d ) Luciferase activity in TLR4-HEK293T cells stimulated for 5 h with LPS (10 ng ml −1 ), 24 h after co-transfection with NF-κB-responsive reporters and: ( a ) empty (Control) or the indicated truncated PLZF constructs. See also Supplementary Fig. 5 ; ( b ) PLZF, HDAC1, HDAC2, HDAC3 or NF-κB p50 expression constructs; ( c ) WT or catalytically inactive HDAC3 (Y298H); and ( d ) HDAC3 with NF-κB p50, or PLZF, and all three protein expression constructs combined. ( e , f ) Micrographs showing the interaction between endogenous PLZF and HDAC3 or NF-κB p50 and HDAC3 with p50 or p65 detected as red foci in ( e ) RAW264.7 cells, or ( f ) WT and Zbtb16 −/− BMMs stimulated with LPS (100 ng ml −1 ). Graphs below show a quantitation of the protein interactions detected by PLA from 200 cells (using OLINK). HDAC4 and the IgG are used as controls. Cell nuclei are stained blue by Hoechst dye (scale bar, 10 μm). ( g ) Detection of the dependence of the K277 residue of PLZF for protein association by BiFl using HEK293T cells transfected with WT or mutant (K277R) PLZF tagged with the V2 split Venus fluorophore and either NF-κB p50 or HDAC3 fused with the alternate V1 half of Venus (scale bar, 10 μm). Expression of PLZF is confirmed with an antibody (αGFP) to V2 and used to normalize the level of Venus fluorescence to protein expression in the graph to the right of the micrographs. The complexes being detected are depicted in the schematic shown on the left of the micrographs. ( h ) Demonstration of the dependence of HAT1 expression for the formation of the co-repressor protein complex, by detecting the association between HDAC3 and PLZF, or NF-κB p50 through IP and immunoblot (IB) with the indicated antibodies in THP-1 cells expressing a control (shCONT) or HAT1 -targeting (shHAT1) shRNAs treated with TNF-α (10 ng ml −1 ) for 30 min. All experiments n ⩾ 3, bars represent mean±s.d. * P <0.05, ** P <0.01, and not significant (NS) by Student’s t -test. Full size image To visualize a direct association between endogenous PLZF, HDAC3 and NF-κB p50, we employed the PLA in the RAW 264.7 mouse macrophage cell line. Resting macrophage cells showed few foci, corresponding to complexes of PLZF-HDAC3 and PLZF-NF-κB p50. However, upon LPS stimulation, foci markedly increased ( Fig. 6e ). Replication of the PLA in the WT and Zbtb16 −/− BMMs confirmed the dependence of PLZF for the association between HDAC3 and NF-κB p50 ( Fig. 6f ). Conversely, formation of the transcriptionally active NF-κB p65-p50 heterodimer was reduced by PLZF ( Fig. 6f ). We also show by bimolecular fluorescence complementation assay that the association between PLZF and HDAC3, or NF-κB p50, each tagged with separate halves of a split Venus fluorophore and expressed in HEK293 cells, was dependent on the K277 residue ( Fig. 6g ). Moreover, we demonstrate by co-IP and immunoblot of each protein constituent in THP-1 cells with normal or reduced HAT1 expression that formation of the PLZF-HDAC3-NF-κB p50 protein complex requires HAT1 expression ( Fig. 6h ). These data identified that NF-κB activity is controlled by a PLZF-HDAC3-NF-κB p50 protein complex that appears to be regulated by acetylation of the K277 residue of PLZF by HAT1. The PLZF-HDAC3-NF-κB p50 complex is a transcriptional repressor We performed chromatin immunoprecipitation (ChIP) studies to link the formation of this protein complex with transcription. These data show that before stimulation, PLZF, NF-κB p50 and HDAC3 associate with the Il-12 and Tnf-α promoters ( Fig. 7 and Supplementary Fig. 6a ). Following treatment of WT BMMs with LPS, HDAC3 is gradually displaced from these promoters, an event that coincides with the binding of NF-κB p65 and the transcriptional co-activator p300. Notably, the disassociation of HDAC3 and concomitant recruitment of NF-κB p65 and p300 occurred more rapidly following LPS stimulation in the absence of PLZF ( Fig. 7a,c ). Co-operativity between PLZF, HDAC3 and NF-κB p50 was further supported by sequential ChIP (Re-ChIP). We found that the Il-12 promoter retained bound NF-κB p50 and HDAC3, even after LPS treatment, in the WT but not Zbtb16 −/− BMMs ( Fig. 7b ). By contrast, greater quantities of active NF-κB p65 and p50 complex could be enriched from the Il-12 promoter in the Zbtb16 −/− compared with the WT cells upon LPS stimulation. To precisely match the kinetics by which the transcription factors associate with each other and the DNA, we conducted quantitative ChIP PCR analysis of the Tnf-α gene promoter ( Fig. 7c and Supplementary Fig. 6a,b ). These data demonstrate that the reciprocal loss of HDAC3 and enhanced recruitment of NF-κB p65 and p300 coincide with the observed formation of the either activating or repressor complexes in the Zbtb16 −/− compared with the WT BMMs. 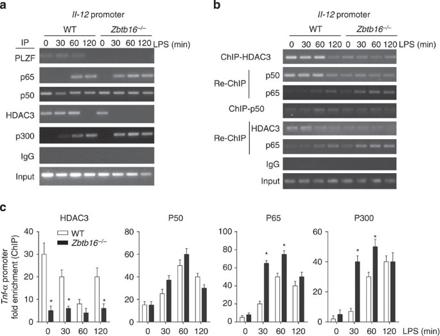Figure 7: The PLZF-HDAC3-NF-κB p50 complex is a transcriptional repressor. (a–c) Measure of transcriptional factor binding to gene promoters by detecting PCR amplicons from theIL-12p40andTNF-αpromoters after (a) ChIP of products with anti-PLZF, -NF-κB p65, -p50, -HDAC3, -p300 or, as a control, an IgG antibody, from WT andZbtb16−/−BMMs treated with LPS (10 ng ml−1) for the times indicated. (b) Re-ChIP of products initially IP from WT andZbtb16−/−BMMs treated with LPS (10 ng ml−1) for the times indicated. The initial IP used anti-HDAC3 or -NF-κB p50 antibodies that were then Re-ChIP with anti-NF-κB p50, -p65 or -HDAC3, as indicated. The amplicons from the total lysates for each promoter are shown at the bottom (Input). (c) Graphs quantitating sequence tags from theTnf-αpromoter enriched by ChIP with anti-HDAC3, -NF-κB p50, -p65 and -p300 antibodies from WT andZbtb16−/−BMMs treated with LPS (10 ng ml−1) for the times indicated. The graphs show the mean±s.e.m. (*P<0.05 by Student’st-test,n=3). Figure 7: The PLZF-HDAC3-NF-κB p50 complex is a transcriptional repressor. ( a – c ) Measure of transcriptional factor binding to gene promoters by detecting PCR amplicons from the IL-12p40 and TNF-α promoters after ( a ) ChIP of products with anti-PLZF, -NF-κB p65, -p50, -HDAC3, -p300 or, as a control, an IgG antibody, from WT and Zbtb16 −/− BMMs treated with LPS (10 ng ml −1 ) for the times indicated. ( b ) Re-ChIP of products initially IP from WT and Zbtb16 −/− BMMs treated with LPS (10 ng ml −1 ) for the times indicated. The initial IP used anti-HDAC3 or -NF-κB p50 antibodies that were then Re-ChIP with anti-NF-κB p50, -p65 or -HDAC3, as indicated. The amplicons from the total lysates for each promoter are shown at the bottom (Input). ( c ) Graphs quantitating sequence tags from the Tnf-α promoter enriched by ChIP with anti-HDAC3, -NF-κB p50, -p65 and -p300 antibodies from WT and Zbtb16 −/− BMMs treated with LPS (10 ng ml −1 ) for the times indicated. The graphs show the mean±s.e.m. (* P <0.05 by Student’s t -test, n =3). Full size image Together, these data demonstrate that a co-repressor complex consisting of PLZF, NF-κB p50 and HDAC3 limits the production of inflammatory cytokines in response to innate immune cell signalling. This co-repressor complex assembles on the promoters of NF-κB-regulated genes, to the exclusion of activating transcriptional complexes (NF-κB p50-p65), following acetylation of the K277 residue of PLZF by HAT1. HAT1 is activated during TLR or TNFR signalling by CaMK2 activity. Accordingly, diminishing the activity of CaMK2 with a pharmacological inhibitor, knocking down the expression of the kinase, HAT1 and PLZF, mutating specific amino acids that are covalently modified on PLZF (K277) or HAT1 (S361) in cells, or genetically ablating PLZF in mice all curtail the usual control of the production of inflammatory cytokines. Our studies identify a novel cell signalling pathway encompassing acetylation that is of significance to the immune response. To date, the activity of protein kinases and their cognate phosphatases have formed the core of our understanding of cell signal transduction. Although it has come to be appreciated that protein acetylation is as significant as phosphorylation, there have been few expositions of the biological consequences of acetylation [1] . Previously, acetylation of PLZF by p300 had been shown to promote the association of the transcription factor with gene promoters [7] . CBP/p300 had also been demonstrated to modulate the transcriptional activity of the tumour-suppressor p53 (ref. 18 ), and acetylation of the signal transducer and activator of transcription 2 and IRF9 to control cytokine signalling [19] . In addition, the activity of the α-tubulin acetyltransferase (α-TAT) is important for the formation of microtubules. HAT1 had not previously been identified to acetylate non-histone substrates. Recognition of PLZF as an unconventional substrate for HAT1 delineates a cell signalling pathway that, by also encompassing the kinase response, links engagement of cell surface receptors with the transcriptional responses that is distinct from the previously defined role of HAT1 in histone-3 and -4 acetylation. The signalling pathway we identify here may also account for desensitization to persistent noxious stimuli, with the conferred cross-tolerance between TLR, TNFR and IL receptors potentially co-ordinated by convergent engagement of the IL-1 receptor-associated kinase that recruits CaMK2 (ref. 12 ), thereby activating HAT1 to form the PLZF co-repressor complex. It remains to be demonstrated that the CaMK2-dependent activation is mediated by direct phosphorylation of HAT1. Interestingly, CaMK2 has previously been demonstrated to initially advance the production of inflammatory transcripts from TLR and other innate immune receptors [11] . Hence, the kinase appears to immediately promote the response but then initiates processes to restrain ongoing inflammation. Part of the PLZF-dependent repressive mechanism we delineate here had been revealed by the identification of translocation mutations between the retinoic acid receptor α (RARα) and the N-terminal half of PLZF in acute promyelocytic leukaemias [20] . The chimeric proteins formed between PLZF and RARα are transforming as the oncoprotein antagonizing the normal function of the RARα by PLZF-dependent recruitment of the nuclear co-repressor HDAC complex [21] , [22] . We demonstrate that PLZF functions via an analogous mechanism to repress NF-κB-dependent transcription. These results are consistent with the report that in CD4 + T cells, PLZF represses the NF-κB-regulated genes encoding IL-2 and IFN-γ [23] . Inflammatory responses are critical to survival and must be tightly regulated to ensure appropriate immune protection without damage to the host. The inducible NF-κB protein complex constitutes the principal immediate response to a broad range of infectious stimuli. NF-κB does not function in isolation and a variety of transcriptional co-factors modulate its activity. Identification of these separate co-factors and their role in modulating NF-κB activity has the potential to identify strategies to control a harmful immune response. Mice and reagents All mice used in experiments were treated in accordance with practices approved by the Monash University, Monash Medical Centre Animal Ethics Committee (Melbourne, Australia), as obligated by the Australian Code of Practice for the Care and Use of Animals for Scientific Purposes, in compliance with standards mandated by the Australian National Health and Medical Research Council and National Institutes of Health. Mice were bred in high-barrier specific pathogen-free conditions on a C57BL/6 genetic background. PLZF ( Zbtb16 −/− ), NF-κB p65 ( RelA −/− :Tnfr1 −/− ) and c-Rel (Rel −/− :Tnfr1 −/− ) mice of either gender were killed for bone marrow between 7 and 10 weeks of age [24] , [25] . To circumvent the embryonic lethality of RelA-deficient mice, we generated haematopoietic chimeras using E13 fetal livers as a source of haematopoietic stem cells. Fetal liver chimeras were made by engrafting lethally irradiated Ly5.1 + C57BL/6 mice with embryonic day 13 fetal-derived haematopoietic stem cells (Ly5.2 + ) from rela −/− mice as described previously [26] . Eight weeks post engraftment bone marrow was isolated from chimera mice, stained with PE-conjugated anti-Ly5.1 antibodies and the Ly5.1 − fraction was sorted using a FACS Aria cell sorter. Recoveries for Ly5.2+ ( rela −/− ) bone marrow cells were ⩾ 95%. To generate BMMs, cells were flushed from the femur and tibia bones and cultured in L929-conditioned medium to differentiate as described previously [5] , [27] . Mouse macrophages were transfected by nucleofection with a Mouse Macrophage Nucleofector kit (Amaxa). WT and mutant (K271R+K277R) PLZF constructs were expressed in BMM by transformation of the infectious recombinant retrovirus based upon the pRP-HA-mCitrine plasmid. LPS, polyI:C, imiquimod and TNF-α were purchased from Invivogen. Mice were injected with 20 mg kg −1 LPS. The Wilcoxon signed-rank test was used to compare survival in the two groups of mice. The BAY11-7085 (Sigma) and KN-93 (Cayman Chemicals) inhibitors were used at 20 μM concentration. Quantitative real-time PCR Quantitative-PCR (Q-PCR) was done in triplicate on an Applied Biosystems 7700 Prism real-time PCR machine with TaqMan probes for Il-6 , Il-12 , Tnf-α and Rsad2 (Applied Biosystems). Expression of mRNA was normalized to the expression of 18S ribosomal RNA by the change in cycling threshold (Δ C T ) method and calculated based on 2 −ΔCT . Results are expressed as relative gene expression for each target gene. ChIP assay After cell fixing and cell lysis, DNA was broken up by using the Covaris sonicator; equal amounts of lysates were used for IP of chromatin with Dynabeads Protein A (Invitrogen) and 2 μg of antibody against: PLZF (Calbiochem), NF-κB p65 (sc-372, Santa Cruz; or 06-418, Millipore), p300 (05-257, Millipore), p50 (sc-114), HDAC3 (sc-8138), IRF3 (sc-9028) or IgG (sc-372 or sc-2434), as a control (all purchased from Santa Cruz). After washing with salt buffer, LiCl buffer and Tris-EDTA (TE) buffer, the Dynabeads Protein A complexes were mixed with 10% Chelex-100 slurry, boiled for 10 min and treated with proteinase K for 2 h. The beads were then boiled again for 10 min, and following centrifugation, the supernatant was collected and used for ChIP PCR. Sonicated chromatin (1%) was used as a positive control to ensure equal input. All quantitative ChIP PCR data were normalized to those of IgG control samples and fold enrichments were calculated. The presence of the target gene promoter sequences in both the input DNA and the recovered DNA immunocomplexes was detected by Q-PCR. PCR for Tnf-α , Il-6 and Il-12p40 was performed using a SYBR Green PCR master mix (AP Biotech) on an iCycler iQ PCR machine (Bio-Rad). Primer pairs (amplifying a PCR product spanning the NF-κB site) were: 5′- CCCCAGATTGCCACAGAATC -3′ and 5′- CCAGTGAGTGAAAGGGACAG -3′ for the Tnf-α promoter; 5′- CAGCAGCCAACCTCCTCTAA -3′ and 5′- CTGTGAGCGGCTGTTGTAGA -3′ for the Il-6 promoter; 5′- AGTATCTCTGCCTCCTTCCTT -3′ and 5′- GCAACACTGAAAACTAGTGTC -3′ for the Il-12 promoter; and as negative control 5′- AGCTCCAAGAAAGGACGAACAT -3′ and 5′- GCCCTGTAGGTGAGGTTGATCT -3′ for IFN-β promoter. For Re-ChIP, the precipitated Dynabeads Protein A complexes were washed with TE, then suspended in TE with dithiothreitol and incubated at 37 °C for 30 min. Following centrifugation at 800 g for 2 min, the supernatant was diluted for the next round of ChIP. Assay of luciferase reporter gene expression The total amount of plasmid DNA transfected was equalized by the addition of empty control vector. After 24 or 36 h, cells were left untreated or were treated with LPS, at 10 ng ml −1 for the BMM or 100 ng ml −1 for the TLR4-HEK293 and RAW cells, and polyI:C 25 μg ml −1 and TNF-α at 10 ng ml −1 for 5 h. Luciferase activity was measured with a dual-luciferase reporter assay system according to the manufacturer’s instructions (Promega) in a FLUOstar Optima plate reader (BMG Labtech). Data were normalized for nonspecific expression by the division of firefly luciferase activity with that of renilla luciferase. Immunoprecipitation and western blotting analysis For IP, cells were lysed with triple detergent lysis buffer and incubated with each antibody. Nuclear and cytoplasmic fractionation was performed using NE-PER nuclear protein extraction kit (Pierce) according to the manufacturer's instructions. Antibody complexes were isolated with protein A/G–agarose beads (Pharmacia Biotech), fractionated by SDS/PAGE, transferred to polyvinylidene fluoride membrane and detected by western blotting using: phosphorylation-specific antibodies to ERK (phospho-Thr202-Tyr204, E10), JNK (phospho-Thr183-Tyr185, G9), p38 (phospho-Thr180-Tyr182, 9211) and CaMK2 (phosphor-T286, 3361) (from Cell Signaling Technology); anti-acetylated lysine residue and anti-CaMK2 (3361) antibodies (Cell Signaling Technology); anti-β-actin (sc-130656), -IκBa (sc-371), -NF-κB p65 (sc-109) and -NF-κB p50 (sc-1190) antibodies (Santa Cruz Biotechnology); anti-FLAG (M2) and anti-Myc antibodies (Sigma-Aldrich); anti-HAT1 antibody (ab61225) (Abcam); and anti-GFP antibody (clone 7.1 and 13.1) (Roche). Targeted proteins were detected and quantified on an Odyssey (LI-COR Biosciences) infrared imaging system. Images have been cropped for presentation. Full-size images are presented in Supplementary Figs 7–9 . Immunofluorescence analysis and PLA The cells were incubated with a 1 in 1,000 dilution of primary antibodies against: NF-κB p65, NF-κB p50, HDAC3 (from Santa Cruz), HAT1 (Abcam) or PLZF (Calbiochem). After washing, primary antibodies were detected with the appropriate Alexa Fluor-conjugated secondary antibodies (Invitrogen). Nuclei were visualized with Hoechst 33258 (Invitrogen). The PLA used mouse anti-PLZF and rabbit anti-HDAC3, rabbit anti-NF-κB p50 or rabbit anti-HAT1. The interaction of PLZF with NF-κB p50, HDAC3 and HAT1 was assessed using a Duolink PLA assay kit following the manufacturer’s protocol (Olink Bioscience). Briefly, sections/cells were fixed with 4% paraformaldehyde for 15 min. The slides were washed twice with PBS, blocked for 1 h at room temperature with 2% BSA in PBS containing 0.1% Triton X-100, followed by incubation with the specified antibody pairs overnight at 4 °C. PLA was performed using anti-PLZF and IgG, or anti-PLZF and anti-HDAC4 antibodies as negative controls. Detection of the association between endogenous HDAC3 and NF-κB p50 or p65 and NF-κB p50 was performed using the relevant mouse or rabbit antibodies. Images were acquired by confocal microscopy (Nikon-C1) and the protein interactions quantitated from 200 cells (using OLINK). Detection of protein associations by BiFl used HEK293T cells transfected with WT or mutant (K277R) PLZF tagged with the V2 split Venus fluorophore and either NF-κB p50 or HDAC3 fused with the alternate half of Venus (V1). Expression of PLZF is confirmed with an antibody (αGFP) to V2. EMSA and TransAM NF-κB Nuclear extracts were incubated with [γ- 32 P]dATP-radiolabelled oligonucleotides containing a consensus binding site for NF-κB/Rel family with homodimeric and heterodimeric complexes (5′- AGTTGAGGGGACTTTCCCAGGC -3′; Santa Cruz Biotechnology). DNA-protein complexes were resolved from free labelled DNA by electrophoresis through native 4% (wt/vol) polyacrylamide gels and the dried gels were analysed by autoradiography. NF-κB p65 DNA-binding assays were performed according to the protocols described in the TransAM® NF-κB p65 kit (Active Motif). Statistical analysis All statistical analyses were performed with Graphpad Prism software. Differences in survival rates were assessed by the log-rank test, using the unpaired, two-tailed t -test to analyse the data and generate P values. P values of less than 0.05 were considered significant. How to cite this article: Sadler, A. J. et al . The acetyltransferase HAT1 moderates the NF-κB response by regulating the transcription factor PLZF. Nat. Commun. 6:6795 doi: 10.1038/ncomms7795 (2015).